A highly efficient cocaine-detoxifying enzyme obtained by computational design Compared with naturally occurring enzymes, computationally designed enzymes are usually much less efficient, with their catalytic activities being more than six orders of magnitude below the diffusion limit. Here we use a two-step computational design approach, combined with experimental work, to design a highly efficient cocaine hydrolysing enzyme. We engineer E30-6 from human butyrylcholinesterase (BChE), which is specific for cocaine hydrolysis, and obtain a much higher catalytic efficiency for cocaine conversion than for conversion of the natural BChE substrate, acetylcholine (ACh). The catalytic efficiency of E30-6 for cocaine hydrolysis is comparable to that of the most efficient known naturally occurring hydrolytic enzyme, acetylcholinesterase, the catalytic activity of which approaches the diffusion limit. We further show that E30-6 can protect mice from a subsequently administered lethal dose of cocaine, suggesting the enzyme may have therapeutic potential in the setting of cocaine detoxification or cocaine abuse. As well known, naturally occurring enzymes are exceptional catalysts that recruit their substrates to a precisely defined active site with precisely aligned catalytic amino-acid residues and an ideal protein environment for rapid chemical transformation and, thus, accelerate chemical reactions under mild conditions. For example, acetylcholinesterase (AChE) has been well known as the most efficient hydrolytic enzyme, with the catalytic activity for neurotransmitter acetylcholine (ACh) approaching the limit allowed by the diffusion of the substrate [1] . Typically, the catalytic activities for naturally occurring enzymes are within three orders of magnitude of the diffusion limit [2] . It is highly desired for drug discovery, drug delivery, therapeutic development, chemical engineering, natural product production, chemical defence, green chemistry and biomediation of xenobiotic pollutants to have the ability to design new enzymes with the catalytic activities comparable to those of naturally occurring enzymes. Recently reported studies have demonstrated that computational enzyme design can lead to discovery of active enzymes [2] , [3] , [4] , [5] , [6] , [7] , [8] , [9] , [10] , [11] , [12] , [13] , [14] . However, computationally designed enzymes to date are much less efficient, with the catalytic activities being more than six orders of magnitude from the diffusion limit [2] . Here we report our successful computational design of a highly efficient enzyme with the catalytic efficiency specific for cocaine detoxification comparable to that of an evolutionarily perfect enzyme [1] , that is, AChE (for ACh) known as the most efficient naturally occurring esterase. Cocaine is recognized as the most reinforcing one of widely abused drugs in stimulating the reward pathway of the brain and teaching the user to take it again [15] , [16] , [17] . There is no FDA-approved medication specific for cocaine. An ideal anticocaine medication would be to accelerate cocaine metabolism producing biologically inactive metabolites [18] . Hydrolysis of cocaine at the benzoyl ester group produces ecgonine methyl ester and benzoic acid that are all biologically inactive [15] . As well known, an effective esterase should have some essential residues aligned to form an active site consisting of a catalytic triad/diad (such as Ser-His-Asp or Ser-His-Glu as a triad) and an oxyanion hole with hydrogen bond donors [14] , [19] , [20] . The catalytic triad may initialize the nucleophilic attack on the carbonyl carbon of the ester group, while the oxyanion hole can form hydrogen bonds with the carbonyl oxygen of the ester group and, thus, stabilizes the transition states during the reaction process. In fact, numerous proteins have these essential residues. For example, all serine hydrolases, including AChE and its cousin butyrylcholinesterase (BChE) [19] , [20] , have the catalytic triad and oxyanion hole, and one may start from a serine hydrolase as the protein scaffold to design a cocaine hydrolase capable of hydrolysing cocaine in the way shown in Fig. 1 . 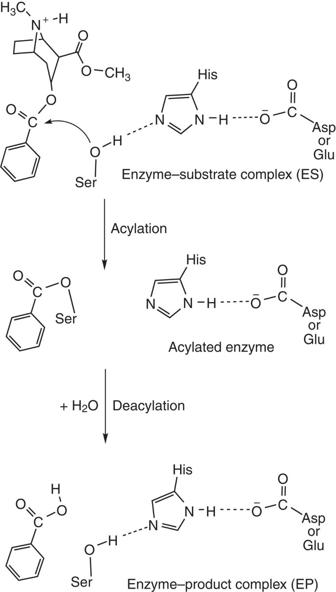Figure 1:(−)-Cocaine hydrolysis in a desired serine hydrolase that has a catalytic triad consisting of three essential amino-acid residues (Ser, His and Asp/Glu) and an oxyanion hole consisting of H-bond donors (not shown) surrounding the carbonyl oxygen of the substrate.  Figure 1: (−)-Cocaine hydrolysis in a desired serine hydrolase that has a catalytic triad consisting of three essential amino-acid residues (Ser, His and Asp/Glu) and an oxyanion hole consisting of H-bond donors (not shown) surrounding the carbonyl oxygen of the substrate. Full size image Human BChE [21] represents an ideal protein scaffold to design the desired cocaine hydrolase because it is highly thermostable (with a half-life of ~12 days in humans) and a safe enzyme for humans; no adverse effects have been observed for using a wild-type or mutant BChE in humans [22] , [23] . ACh is the only natural substrate for AChE and BChE in human body [20] . Wild-type BChE has a low catalytic efficiency against naturally occurring (−)-cocaine ( k cat =4.1 min −1 , K M =4.5 μM and k cat / K M =9.1 × 10 5 min −1 M −1 ) [24] , too low to be used as a therapeutic agent. In general, the catalytic efficiency of an enzyme for a substrate reaction is represented by k cat / K M , that is, the ratio of the catalytic rate constant ( k cat ) to the Michaelis–Menten constant ( K M ). Previous computational enzyme design has generated BChE mutants with a significantly improved catalytic efficiency for (−)-cocaine hydrolysis [19] , [20] , [24] , [25] , [26] , [27] , [28] . The most successful previous design (that is, the A199S/S287G/A328W/Y332G mutant, with k cat =3,060 min −1 , K M =3.1 μM and k cat / K M =9.9 × 10 8 min −1 M −1 ) (refs 26 , 29 ) was proposed [30] for future clinical trials in humans. However, even if the clinical trial is successful, the enzyme therapy using this BChE mutant in practical clinical use would be very expensive due to the need of a high dose (~5 mg kg −1 ) of the enzyme. Thus, it is highly desired to further improve the catalytic activity of the enzyme against (−)-cocaine, to decrease the required dose of the enzyme and, thus, the costs of the enzyme therapy. The higher the catalytic activity, the lower the dose required for the effective treatment of cocaine abuse. On the other hand, it is considerably more challenging for computational enzyme redesign to further improve the catalytic activity of an enzyme when its catalytic activity is already high. By using a two-step computational design approach, in the present study, we have successfully engineered a cocaine-detoxifying enzyme E30-6 from human butyrylcholinesterase (BChE), which is specific for cocaine hydrolysis, with a catalytic efficiency for cocaine comparable to that of AChE for ACh. We have further demonstrated that E30-6 can protect mice from a subsequently administered lethal dose of cocaine, suggesting the enzyme may have therapeutic potential in the setting of cocaine detoxification or cocaine abuse. Computational design According to previous computational modelling [19] , [26] , [27] of the transition states (TSs) for (−)-cocaine hydrolysis catalysed by various BChE mutants, the experimental catalytic efficiency of the enzyme (BChE or mutant) against (−)-cocaine correlates with the overall strength of all hydrogen bonds (HBs) between the carbonyl oxygen of (−)-cocaine and the oxyanion hole of the enzyme in the transition state (TS1) for the initial step of the enzymatic reaction. Mutations on certain amino-acid residues that are not in the active site may also indirectly perturb the HB distances and, therefore, influence the catalytic activity of the enzyme [19] . The finding of the correlation was based on the use of an empirical hydrogen bonding energy (HBE) equation implemented in AutoDock program suite [31] : HBE( R )≈5 εR 0 12 / R 12 –6 εR 0 10 / R 10 , in which R is the H … O distance in the considered HB and R 0 is the minimum value of the H … O distance for which the HBE equation can be used [26] . It has been known that the total HBE (tHBE) values in other TS’s correlate with the tHBE value in TS1 for the enzymatic hydrolysis [32] , suggesting that a BChE mutant associated with a lower tHBE value in TS1 should also have lower tHBE values in other TS’s for the same reaction. It has also been demonstrated that the tHBE value (a negative value) is proportional to a simplified descriptor, in which R i represents the O … H distance in the i th hydrogen bond between the carbonyl oxygen of (−)-cocaine and the oxyanion hole (consisting of residues G116, G117 and S199) of the enzyme in the TS1 structure. [19] Taking advantage of the above-mentioned correlation, in the present study, we carried out extensive virtual screening of the possible TS1 structures associated with various designs (BChE mutants) in a carefully designed virtual library (see below for the library design) to identify the one with the largest possible value. In the virtual screening, for each design, we only needed to model the TS1 structure giving a value. The virtual screening revealed that the largest value was associated with design E30-6, which is the A199S/F227A/P285A/S287G/A328W/Y332G mutant of human BChE. To confirm the design E30-6 based on the above-mentioned simple correlation relationship, we further performed more sophisticated computational evaluation based on hybrid quantum mechanical/molecular mechanical (QM/MM)-free energy (FE) calculations on E30-6-catalysed hydrolysis of (−)-cocaine to determine the detailed reaction coordinate and free energy change during the enzymatic reaction process. As well known [26] , an ester hydrolysis by a serine hydrolase always consists of the acylation and deacylation of the ester, and the acylation process is rate controlling for (−)-cocaine hydrolysis catalysed by the known BChE mutants in light of both computational and experimental data. Hence, our QM/MM-FE calculations were focused on the acylation process. The QM/MM-FE calculations revealed that the acylation of (−)-cocaine in E30-6 consists of three reaction steps. The initial reaction step is the nucleophilic attack on carbonyl carbon of (−)-cocaine benzoyl ester by hydroxyl group of S198 while the the serine hydroxyl group of S198 transfers a proton to the nitrogen atom of H438 side chain. Then, the (−)-cocaine benzoyl ester bond breaks, with the ester oxygen leaving the carbonyl carbon (the second step), followed by a proton transfer from the nitrogen atom of H438 side chain to the ester oxygen (the third step). Depicted in Fig. 2 are the QM/MM-optimized geometries of the enzyme–substrate (ES) complex, transition states (TSs) and intermediates (INTs) involved in the acylation process, along with the free energy changes during the acylation reaction process (ES→TS1→INT1→TS2→INT2→TS3→INT3). This three-step acylation mechanism is remarkably different from the well-known two-step acylation mechanism of other ester hydrolysis reactions in serine hydrolases. According to the well-known two-step acylation mechanism, the ester bond breaking and the proton transfer to the ester oxygen are a concerted process. 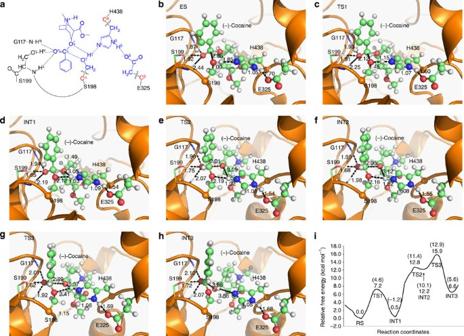Figure 2: Geometries and free energy profile obtained during the acylation stage of (−)-cocaine hydrolysis in E30-6. (a) Division of the QM-MM system: all atoms in blue belong to the QM subsystem in the QM/MM calculations. Three boundary carbon atoms (Cαor Cβ, coloured in red) were treated with as the pseudobond parameters. All other atoms belong to the MM subsystem. (b–h) Key states of the reaction system in the acylation stage, including the prereactive enzyme–substrate (ES) complex, first transition state (TS1), first intermediate (INT1), second transition state (TS2), second intermediate (INT2), third transition state (TS3) and third (final) intermediate (INT3). The geometries were optimized at the QM/MM(B3LYP/6-31G*:AMBER) level. The non-polar hydrogen atoms of the oxyanion hole are not shown for clarity. Some key distances in the figure are given in Å. Carbon, oxygen, nitrogen and hydrogen atoms are coloured in green, red, blue and white, respectively. The backbone of the protein is rendered as a cartoon and coloured in orange. The QM atoms are represented in the ball-and-stick style, and the surrounding residues rendered in the stick style. (i) Free energy profile determined by performing the QM/MM-FE calculations at the MP2/6-31+G*:AMBER level excluding the zero-point vibrational and thermal corrections for the QM subsystem. The values in parentheses are relative free energies including the zero-point and thermal corrections for the QM subsystem. Figure 2: Geometries and free energy profile obtained during the acylation stage of (−)-cocaine hydrolysis in E30-6. ( a ) Division of the QM-MM system: all atoms in blue belong to the QM subsystem in the QM/MM calculations. Three boundary carbon atoms (C α or C β , coloured in red) were treated with as the pseudobond parameters. All other atoms belong to the MM subsystem. ( b – h ) Key states of the reaction system in the acylation stage, including the prereactive enzyme–substrate (ES) complex, first transition state (TS1), first intermediate (INT1), second transition state (TS2), second intermediate (INT2), third transition state (TS3) and third (final) intermediate (INT3). The geometries were optimized at the QM/MM(B3LYP/6-31G*:AMBER) level. The non-polar hydrogen atoms of the oxyanion hole are not shown for clarity. Some key distances in the figure are given in Å. Carbon, oxygen, nitrogen and hydrogen atoms are coloured in green, red, blue and white, respectively. The backbone of the protein is rendered as a cartoon and coloured in orange. The QM atoms are represented in the ball-and-stick style, and the surrounding residues rendered in the stick style. ( i ) Free energy profile determined by performing the QM/MM-FE calculations at the MP2/6-31+G*:AMBER level excluding the zero-point vibrational and thermal corrections for the QM subsystem. The values in parentheses are relative free energies including the zero-point and thermal corrections for the QM subsystem. Full size image As seen in Fig. 2 (I), the free energy barrier calculated for the initial step of the reaction is only 4.5 kcal mol −1 (after the zero-point and thermal corrections to the Gibbs free energies). The TS1 structure for E30-6 is so stable that the free energy of TS1 is significantly lower than those of TS2 and TS3. For this reaction, the overall free energy barrier for the entire acylation reaction process is actually associated with the free energy change (~14.1 kcal mol −1 ) from INT1 to TS3 (after the zero-point and thermal corrections to the Gibbs free energies). The calculated overall free energy barrier of ~14.1 kcal mol −1 would predict that the k cat value for this design for (−)-cocaine hydrolysis should be in the order of ~10 4 min −1 , according to the well-known conventional transition state theory (CTST) [33] . In vitro activities of the enzymes According to the above computational prediction, we produced E30-6 and 12 other designs listed in Table 1 through site-directed mutagenesis, protein expression, purification, active site titration and enzyme activity assays. The initial activity assays (using 1 mM (−)-cocaine) determined the relative V max values against (−)-cocaine as summarized in Table 1 , revealing that design E30-6 has the largest V max value against (−)-cocaine. The best design E30-6 was examined further by performing enzyme activity assays in vitro and in vivo . Table 1 Kinetic parameters of selected designs for (−)-cocaine hydrolysis, determined by the initial in vitro activity assays. Full size table Michaelis–Menten kinetics of the enzymatic (−)-cocaine hydrolysis at the benzoyl ester group and that of enzymatic ACh hydrolysis were determined by performing the sensitive radiometric assays using [ 3 H]( −)-cocaine and [ 3 H]ACh with varying concentrations of the substrates. On the basis of in vitro kinetic analysis (see Fig. 3 ), k cat =14,600 min −1 , K M =3.65 μM and k cat / K M =4.0 × 10 9 min −1 M −1 for (−)-cocaine hydrolysis in E30-6, whereas k cat =8710, min −1 , K M =54.7 μM and k cat / K M =1.6 × 10 8 min −1 M −1 for ACh hydrolysis in E30-6. The obtained kinetic parameters are summarized in Table 2 in comparison with known kinetic parameters for ACh hydrolysis in BChE and AChE. The kinetic data show that, for (−)-cocaine hydrolysis in E30-6, k cat is significantly larger and K M is significantly smaller compared with ACh hydrolysis in E30-6. As a result, the catalytic efficiency ( k cat / K M ) of E30-6 for (−)-cocaine is higher than that for ACh by ~25-fold. 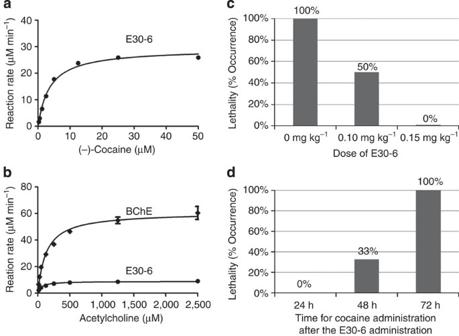Figure 3: Kinetic characterization andin vivoeffects of E30-6. The reaction rates were determined by using sensitive radiometric assays using [3H](−)-cocaine. (b) Plots of measured reaction rates vs the ACh concentration; the enzyme was E30-6 or human BChE. The reaction rates were determined by using sensitive radiometric assays using [3H]ACh. All of the assays were performed in triplicate, and the data were present with error bars (s.e.m.). (c) Effects of E30-6 in the protection of mice against the acute toxicity of a lethal dose of cocaine (180 mg kg−1, i.p.). The enzyme (E30-6) was administered intravenously (i.v.) 1 min before intraperitoneal administration of cocaine 180 mg kg−1(LD100). Each data point represents the percentage of mice (n=6 for each dosing condition) exhibiting cocaine-induced lethality. (d) Duration of the protective effects provided by E30-6. A separate set of mice (n=6) were challenged with 180 mg kg−1cocaine (i.p.) every 24 h (that is, 24 h, 48 h and 72 h, until no mice survived) after the administration of 3 mg kg−1E30-6 (i.v.). Figure 3: Kinetic characterization and in vivo effects of E30-6. The reaction rates were determined by using sensitive radiometric assays using [ 3 H](−)-cocaine. ( b ) Plots of measured reaction rates vs the ACh concentration; the enzyme was E30-6 or human BChE. The reaction rates were determined by using sensitive radiometric assays using [ 3 H]ACh. All of the assays were performed in triplicate, and the data were present with error bars (s.e.m.). ( c ) Effects of E30-6 in the protection of mice against the acute toxicity of a lethal dose of cocaine (180 mg kg −1 , i.p.). The enzyme (E30-6) was administered intravenously (i.v.) 1 min before intraperitoneal administration of cocaine 180 mg kg −1 (LD 100 ). Each data point represents the percentage of mice ( n =6 for each dosing condition) exhibiting cocaine-induced lethality. ( d ) Duration of the protective effects provided by E30-6. A separate set of mice ( n =6) were challenged with 180 mg kg −1 cocaine (i.p.) every 24 h (that is, 24 h, 48 h and 72 h, until no mice survived) after the administration of 3 mg kg −1 E30-6 (i.v.). Full size image Table 2 Kinetic parameters for enzymatic hydrolysis of (−)-cocaine and ACh. Full size table Comparing the measured relative V max values with the calculated values for the designs listed in Table 1 , one can obtain a reasonable (although not perfect) linear correlation between the V max and with the correlation coefficient ( r ) being 0.786 and root-mean-square deviation (RMSD) being 20.7% (see Supplementary Table 1 and Supplementary Fig. 1 for the detailed data). It is well known that native human BChE has a high thermal stability because it mainly exists in the tetramer structure [34] . We examined E30-6 by using a non-denaturing polyacrylamide gel ( Supplementary Fig. 2 ), and the obtained gel indicated that E30-6 also mainly existed in the tetramer structure. In vivo effects of E30-6 On the basis of promising in vitro activity, we further evaluated the potential therapeutic value of E30-6 by using in vivo models. We first tested the potential toxicity of E30-6 itself in mice and did not note any sign of the toxicity during the 3-week observations, suggesting that E30-6 is a safe enzyme. Further, we wanted to know whether E30-6 can effectively protect mice from the acute toxicity of a lethal dose of cocaine (180 mg kg −1 , LD 100 ). As shown in Fig. 3c , for the negative control experiments without administration of the enzyme, intraperitoneal (i.p.) administration of 180 mg kg −1 cocaine produced lethality in all tested mice ( n =6). Pretreatment with E30-6 (that is, 1 min before cocaine administration) dose dependently protected mice against cocaine-induced lethality. In particular, E30-6 at a comparatively low dose of 0.15 mg kg −1 (i.v.) produced full protection in mice after receiving a lethal dose of cocaine (180 mg kg −1 , i.p. ), and E30-6 at a lower dose of 0.10 mg kg −1 (i.v.) produced 50% protection in mice after receiving a lethal dose of cocaine (180 mg kg −1 , i.p.). Hence, 0.15 mg kg −1 may be regarded as the minimum dose of E30-6 required to fully protect mice from the acute toxicity of a lethal dose of cocaine (180 mg kg −1 , i.p.). Further, it is also interesting to examine the duration of the protective effects provided by the enzyme. In previous studies on a bacterial cocaine esterase (CocE) and its thermally stable mutants [35] , [36] , [37] , wild-type CocE or mutant CocE (i.v. dose of 3, 9 or 30 mg kg −1 ) was administered to mice at different time points (30 min, 1 h, 2 h, 3 h, 4 h and 5 h) before cocaine administration (180 mg kg −1 , i.p.) [37] , allowing to estimate the time required to reach 50% lethality (LT 50 ) for a given dose of enzyme. The data revealed that pretreatment (at 30 min or longer) with 3 mg kg −1 (or 0.1 mg per mouse) wild-type or any mutant CocE was ineffective against a lethal dose of cocaine (180 mg kg −1 , i.p. ), suggesting that LT 50 <30 min with 3 mg kg −1 wild-type or any mutant CocE tested. Pretreatment with a larger enzyme dose (9 or 30 mg kg −1 ) was effective. At the highest dose tested (30 mg kg −1 or 1 mg per mouse), LT 50 =14 min, 1.8 h and 4.5 h for the wild-type CocE, T172R CocE and T172R/G173Q CocE, respectively [37] . For comparison, in the present study, a separate set of mice ( n =6) were first administered with 3 mg kg −1 E30-6 (i.v. ), and then challenged with a lethal dose of cocaine (180 mg kg −1 , i.p.) every 24 h (that is, 24 h, 48 h and 72 h) until no mice survived. It turned out that all of mice survived after the first cocaine challenge at 24 h, four mice (67%) survived after the second cocaine challenge at 48 h and no mice survived after the third cocaine challenge at 72 h; see Fig. 3d . The data in Fig. 3d suggest that LT 50 >48 h with 3 mg kg −1 E30-6. The computationally designed new mutations on BChE significantly improved the catalytic activity for (−)-cocaine through enhancing the overall hydrogen bonding between the carbonyl oxygen of (−)-cocaine and the oxyanion hole of the enzyme in the transition state. However, the new mutations have not produced new hydrogen bonds in the transition state. Instead, the new mutations indirectly influence the existing hydrogen bonds between the carbonyl oxygen of (−)-cocaine and the oxyanion hole (residues G116, G117 and S199) in the transition states, thus further stabilizing the transition state and improving the catalytic activity for (−)-cocaine. It should be noted that we have not solved an X-ray crystal structure of enzyme E30-6. Although obtaining an X-ray crystal structure of the transition state for (−)-cocaine hydrolysis in E30-6 would be very challenging, solving a co-crystal structure of E30-6 with a stable analogue of the transition state would be an important future direction for further understanding the improved activity of the enzyme. On the basis of kinetic data summarized in Table 2 , E30-6 has a high specificity for (−)-cocaine over ACh, because the catalytic efficiency ( k cat / K M ) of E30-6 for (−)-cocaine is higher than that for ACh by ~25-fold. Hence, E30-6 is truly qualified to be called a cocaine hydrolase. Such a true cocaine hydrolase dose dependently protected mice against cocaine-induced lethality. All of the in vivo data illustrate that E30-6 may have potential for cocaine detoxification in therapeutic treatment of cocaine abuse. For further demonstration of a therapeutic application of the enzyme in cocaine detoxification treatment, one would also need to develop a feasible animal model in which the enzyme is administered after cocaine administration. Development of such an animal model is our future direction. In addition, the successful design of a highly efficient cocaine hydrolase also demonstrates a promising future of computational enzyme redesign. Compared with ACh hydrolysis in native BChE and AChE, E30-6 has a significantly smaller K M value because of the significantly higher binding affinity, although it has a lower k cat value. As a result, the catalytic efficiency ( k cat / K M =4.0 × 10 9 min −1 M −1 ) for (−)-cocaine hydrolysis in E30-6 is significantly higher than that ( k cat / K M =4.1 × 10 8 min −1 M −1 ) for ACh hydrolysis in BChE [38] and comparable to that ( k cat / K M =7.8 × 10 9 min −1 M −1 ) for ACh hydrolysis in AChE [39] . AChE has been well-known as the most efficient hydrolytic enzyme, with the catalytic activity for ACh approaching the diffusion limit, and, for this reason, AChE has been recognized as an evolutionarily perfect enzyme [1] . Hence, computational design may be performed to engineer an enzyme with a catalytic efficiency comparable to that of the fastest naturally occurring enzyme. The current computational design has led to discovery of a highly efficient enzyme (E30-6 engineered from human BChE) specifically for cocaine detoxification in vitro and in vivo , with the catalytic efficiency for (−)-cocaine much higher than that for the natural substrate (ACh) of human BChE. The catalytic efficiency of E30-6 for (−)-cocaine hydrolysis is comparable to that of the well-known most efficient hydrolytic enzyme AChE for ACh, suggesting that computational enzyme redesign is promising for design of highly efficient enzymes in practical applications. General computational design strategy Our computational enzyme redesign consisted of two steps. The first step was based on the efficient transition-state modelling (energy minimization) using a classical force field using our previously described strategy (described briefly below) [26] . The efficient transition-state modelling allowed us to virtually screen all possible BChE mutants in a carefully designed virtual library for their relative values. The virtual library design started from the A199S/S287G/A328W/Y332G mutant of human BChE and considered further mutations on other amino-acid residues within 20 Å from substrate (−)-cocaine bound in the mutant, including possible additional single, double and triple mutations on the other residues. Thus, included in the virtual library were a number (~6.7 × 10 4 ) of possible pentuple, hextuple and septuple mutants of human BChE. The theoretically identified best BChE mutant (with the largest possible value in the TS1 structure) was examined further by performing the more sophisticated and more time-consuming QM/MM-FE calculations in the next step. A script file was developed in house to allow the automated virtual screening of all BChE mutants in the designed virtual library. For each BChE mutant in the virtual library, the TS1 structure was energy minimized and analysed for its value. We note that used in our virtual screening is a simplified descriptor associated with tHBE defined above. Such a simplified descriptor only accounts for the effects of the O … H distances on the HBE without accounting for the effects of the hydrogen bond angles. Generally speaking, the hydrogen bond angle would be an important parameter in the HBE calculations when different hydrogen bonds are compared. However, for the specific TS1 structures concerning in this study, all of the mutants examined are expected to have the same hydrogen bonds with the similar hydrogen bond angles. In fact, the mutations examined in this study did only perturb the hydrogen bonding between the carbonyl oxygen of (−)-cocaine and the oxyanion hole (residues G116, G117 and S199) in the transition states. Transition-state modelling using a classical force field Our computational enzyme design started from the transition-state modelling [26] using a classical force field (molecular mechanics). It should be mentioned that, in principle, computational modelling, such as energy minimization or molecular dynamics (MD) simulation, using a classical force field can only simulate a stable structure corresponding to a local minimum on the potential energy surface, whereas a transition state during a reaction process is always associated with a first order saddle point on the potential energy surface. Hence, energy minimization (or MD simulation) using a classical force field cannot directly simulate a transition state without any restraint on the geometry of the transition state. Nevertheless, if we can technically remove the freedom of imaginary vibration in the transition state structure, then the number of the degrees of vibrational freedom (normal vibration modes) for a nonlinear molecule will decrease from 3 N –6. N represents the number of atoms of the system. The transition state structure is associated with a local minimum on the potential energy surface within a subspace of the reduced degrees of vibrational freedom, although it is associated with a first order saddle point on the potential energy surface with all of the 3 N –6 degrees of vibrational freedom. Theoretically, the degree of vibrational freedom associated with the imaginary vibrational frequency in the transition state structure can be removed by appropriately freezing the reaction coordinate. The reaction coordinate corresponding to the imaginary vibration of the transition state is generally characterized by a combination of some key geometric parameters. These key geometric parameters are bond lengths of the transition bonds, that is, the forming and breaking covalent bonds during this reaction step of the enzymatic hydrolysis of cocaine, as seen in Fig. 2 . Thus, we just need to maintain the lengths of the transition bonds during the modelling of a transition state. Technically, we can maintain the lengths of the transition bonds by simply fixing all atoms within the reaction centre, by using some constraints on the transition bonds, or by redefining the transition bonds. It should be pointed out that the purpose of performing such type of computational modelling on a transition state is to examine the change of the protein environment surrounding the reaction centre and the interaction between the reaction centre and the protein environment. We were only interested in the energy-minimized structures, as the total energies calculated in this way are meaningless. The energy-minimized structures can be used for the subsequent evaluation of the values. Specifically, computational modelling of the TS1 structures associated with various designs was based on the TS1 geometry determined in our previously reported molecular modelling and reaction coordinate calculations [32] , [40] , [41] on BChE-catalysed hydrolysis of (−)-cocaine; the modelling started from the X-ray crystal structure [42] deposited in the Protein Data Bank (pdb code: 1POP), and the reaction coordinate calculation was carried out by using a hybrid quantum mechanical/molecular mechanical (QM/MM) approach in which the QM part was treated at the B3LYP/6-31G* level and the MM part was treated by using Amber force field. Starting from the QM/MM-optimized TS1 geometry for BChE-catalysed hydrolysis of (−)-cocaine, Amber9 package [43] was used to model the TS1 structures associated with various designs involved in the present study. All designs evaluated in this study were based on the scaffold of BChE, with the same catalytic triad consisting of S198, H438 and E325. The Amber force field parameters were used for all standard amino-acid residues of the designs, whereas (−)-cocaine and other residues (including S198 and H438) involved in the reaction centre were considered as the non-standard residues and parameterized in the same way as used in our other computational studies [40] . The partial atomic charges of the non-standard residues in the TS1 structures were calculated by using the restricted electrostatic potential protocol implemented in the Antechamber module of the Amber9 package following electrostatic potential (ESP) calculations at ab initio HF/6-31G* level using the Gaussian03 program [44] . For the TS1 structure involved in this study, the system was neutralized and solvated in an orthorhombic box of TIP3P water molecule [45] with a minimum solute-wall distance of 10 Å. The solvent water molecules and counter ions in the solvated system were carefully equilibrated and energy-minimized first, and then the entire system was energy-minimized until convergence by using the Sander module of Amber9 program with a convergence criterion of 0.01 kcal mol −1 Å −1 . For the energy minimization, the steepest descent method was used for the first 1,000 steps and then it was switched to the conjugate gradient method until the convergence was achieved (within 4,000 steps). During the energy minimization on the entire system, only the lengths of the transition bonds (that is, the gradually forming/breaking covalent bonds during the reaction step) were restrained. Specifically, there are three transition bonds in the energy-minimized TS1 structure: partial covalent bond between the carbonyl carbon of (−)-cocaine and the hydroxyl oxygen of S198 side chain (the optimized transition bond length: 2.12 Å); partial covalent bond between the oxygen and hydrogen atoms of the hydroxyl group of S198 side chain (the optimized transition bond length: 1.45 Å); partial covalent bond between the hydroxyl hydrogen of S198 side chain and the nitrogen (N ε ) atom of H438 side chain (the optimized transition bond length: 1.15 Å). The particle mesh Ewald (PME) method [46] was used to treat long-range electrostatic interactions. Ten angstroms was used as the non-bonded cutoff. For the virtual screening, the energy-minimized TS1 structures were used to obtain the key internuclear distances required for evaluating the values. A script file was developed in house to allow automated virtual screening of the mutants for their values. QM/MM-FE calculations All of the QM/MM calculations were performed by a pseudobond QM/MM method [47] , [48] implemented recently in a revised version [28] of the Gaussian03 and Amber8 programs. The QM/MM interface was treated by the pseudobond approach [47] , [48] , in which a seven-valence-electron atom with an effective core potential is constructed to replace the boundary atom of the environment part and to form a pseudobond with the boundary atom of the active part. In QM/MM calculations, all atoms of (−)-cocaine and the side chains of S198, H438 and E325 were considered as the QM atoms, whereas the other atoms were regarded as MM atoms ( Fig. 2a ). The QM/MM calculations were performed by using an iterative minimization procedure at the B3LYP/6-31G*:Amber level, that is, the QM calculations were carried out at the B3LYP/6-31G* level, whereas the MM calculations were carried out by using the Amber force field implemented in the Amber8 program. For QM subsystem, the convergence criterion for geometry optimizations follows the original Gaussian03 defaults; for MM subsystem, the geometry optimization convergence criterion is the RMSD of the energy gradient less than 0.1 kcal mol −1 Å −1 . The iterative restrained optimization procedure [47] was then repeatedly applied to different points along the reaction coordinate, resulting in a minimum energy path. Full QM/MM geometry optimizations at the B3LYP/6-31G*:Amber level followed by vibrational frequency analyses were performed to characterize the reactant, intermediates, transition states and product. The contribution of the QM subsystem fluctuation to the free energy change was then calculated with obtained vibrational frequencies using the harmonic approximation. In addition, single-point energy calculations were carried out at the QM/MM(MP2/6-31+G*:Amber) level for each geometry along the minimum energy path. The free energy changes associated with the QM–MM interaction were determined by the free energy perturbation (FEP) method using a revised version [49] of the Amber8 program. The FEP calculations enabled us to more reasonably determine the relative free energy changes due to the QM–MM interaction. In the FEP calculations, sampling of the MM subsystem was carried out with the QM subsystem frozen at different states along the reaction path. Technically, the final (relative) free energy determined by the QM/MM-FE calculations is the QM part of the QM/MM energy (excluding the Columbic interaction energy between the point charges of the MM atoms and the ESP charges of the QM atoms) plus the relative free energy change determined by the FEP calculations. The time step used in the FEP calculations was 2 fs, and bond lengths involving hydrogen atoms were constrained. In sampling of MM subsystem by MD simulations, the temperature was maintained at 298.15 K. Each window of the FEP calculation consisted of 50 ps of equilibration and 300 ps of sampling. The choice of the 300 ps sampling for each window was based on the observation that there was no noticeable difference between the FEP results obtained from the 300 ps sampling and those from the 500 ps sampling for the rate-determining step of the enzymatic reaction process. Both the forward and backward reaction directions were subjected to the FEP calculations. The final relative free energy was taken as the average of the ‘forward’ and ‘backward’ perturbation results. Enzyme preparation To prepare a new mutant of human BChE, the cDNA for the mutant was constructed starting from the cDNA for the A199S/S287G/A328W/Y332G mutant of human BChE in a pRc/CMV expression plasmid [50] . The site-directed mutagenesis was performed by using the QuikChange method [51] , wherein a pair of complementary mutagenic primers are used to amplify the entire plasmid in a thermocycling reaction using pfu polymerase. For example, the primers used for the F227A mutation are 5′-GCC ATT CTG CAA AGT GGT TCC GCT AAT GCT CCT TGG GCG GTA ACA-3′ (forward primer) and 5′-TGT TAC CGC CCA AGG AGC ATT AGC GGA ACC ACT TTG CAG AAT GGC-3′ (reverse primer). The primers used for the P285A mutation are 5′-GTT GTC CCC TAT GGG ACT GCT TTG GGT GTA AAC TTT GGT CCG ACC-3′ (forward primer) and 5′-GGT CGG ACC AAA GTT TAC ACC CAA AGC AGT CCC ATA GGG GAC AAC-3′ (reverse primer). The polymerase chain reaction (PCR) product was treated with Dpn I endonuclease to digest the parental DNA template. Modified plasmid DNA was transformed into Escherichia coli , amplified and purified. The DNA sequence of the enzyme was confirmed by DNA sequencing. The enzyme was expressed in CHO-S cells (Life Technologies, Grand Island, NY). The CHO-S cells were routinely suspension cultured in serum-free medium according to the manufacturer’s instruction at 8% CO 2 , 37 °C on orbit shaker at 125 r.p.m. The secreted enzyme in the collected culture medium was purified by using affinity chromatography on procainamide-sepharose eluted with 0.2 M procainamide, followed by ion exchange chromatography on DE52 and elution with a NaCl gradient in 20 mM Tris-HCl at pH 7.5. Enzyme activity assays Initial in vitro screening of the enzyme activity against (−)-cocaine was carried out by using a single concentration (1 mM) of (−)-cocaine, assuming that K M <<1 mM such that the enzyme was always saturated by 1 mM (−)-cocaine and the maximum reaction velocity (V max ) was reached for a given concentration [E] of the enzyme. V max = k cat [E]. The relative concentrations of the enzymes were determined by using an enzyme-linked immunosorbent assay (ELISA) [26] , [52] described below. The ELISA buffers used in the present study are the same as those described in literature [26] , [52] . Specifically, the coating buffer was 0.1 M sodium carbonate/bicarbonate buffer (pH 9.5). The washing buffer (PBS-T) was 0.01 M potassium phosphate monobasic/potassium phosphate monohydrate buffer (pH 7.5) containing 0.05% (vol/vol) Tween 20. The diluent buffer (EIA buffer) was potassium phosphate monobasic/potassium phosphate monohydrate buffer (pH 7.5) containing 0.9% sodium chloride and 0.1% bovine serum albumin (BSA). To measure (−)-cocaine and benzoic acid, the product of the enzymatic (−)-cocaine hydrolysis, we used sensitive radiometric assays based on toluene extraction of [ 3 H](−)-cocaine labelled on its benzene ring [24] . In brief, to initiate the enzymatic reaction, 100 nCi of [ 3 H](−)-cocaine was mixed with 100 μl of enzyme solution. For Michaelis–Menten kinetic analysis, the enzymatic reactions proceeded at 37 °C and pH 8 with varying concentrations of (−)-cocaine. The reactions were stopped by adding 200 μl of 0.05 M HCl, which neutralized the liberated benzoic acid while ensuring a positive charge on the residual (−)-cocaine. [ 3 H]benzoic acid was extracted by 1 ml of toluene and measured by scintillation counting. Finally, the measured (−)-cocaine concentration-dependent radiometric data were analysed in terms of the standard Michaelis–Menten kinetics so that the catalytic parameters were determined. The enzyme activity assays with [ 3 H]ACh were similar to the assays with [ 3 H](−)-cocaine. The primary difference was that the enzymatic reaction was stopped by addition of 200 μl of 0.2 M HCl containing 2 M NaCl and that the product was [ 3 H]acetic acid for the ACh hydrolysis. In vivo assays Male CD-1 mice (28 to 33 g) of 5–6 weeks old were ordered from Harlan Laboratories, Inc. (Indianapolis, IN) and were housed in groups of four mice per cage. All mice were allowed ad libitum access to food and water, and were maintained on a 12-h light-dark cycle with lights on at 0630 hours in a room kept at a temperature of 21–22 ° C. Experiments were performed in accordance with the Guide for the Care and Use of Laboratory Animals as adopted and promulgated by the National Institutes of Health. The animal procedures used in this study had been approved by the Institutional Animal Care and Use Committee (IACUC) at the University of Kentucky as part of Protocol #2010-0722. (−)-Cocaine HCl (National Institute on Drug Abuse, Bethesda, MD) was dissolved in sterile water and was administered intraperitoneally at a volume of 0.01 ml g −1 . The purified enzyme E30-6 was diluted to the required concentration in phosphate-buffered saline and administered intravenously at a volume of 0.2 ml per mouse. Cocaine-induced acute toxicity was characterized by the occurrence of lethality. Lethality was defined as cessation of observed movement and respiration. The mouse was placed in a small restraint chamber (Outer tube diameter: 30 mm, Inner tube diameter: 24 mm) that left the tail exposed. The tail was cleansed with an alcohol wipe and a 27G1/2 precision glide needle (Fisher Scientific, Pittsburgh, PA) was inserted into one of the side veins for infusion. The intravenous injection volume of E30-6 or the pure phosphate-buffered saline (the control set) was 0.2 ml per mouse, and it was given 1 min before intraperitoneal administration of cocaine 180 mg kg −1 . To staunch the bleeding, sterile gauze and pressure were applied to the injection site. The protective effects of the enzyme were compared with those of the phosphate-buffered saline. In addition, for testing the duration of the protective effects provided by E30-6, a separate set of mice ( n =6) was challenged with 180 mg kg −1 cocaine (i.p.) every 24 h (that is, 24 h, 48 h and 72 h, until no mice survived) after the administration of 3 mg kg −1 E30-6 (i.v. ). How to cite this article: Zheng, F. et al. A highly efficient cocaine-detoxifying enzyme obtained by computational design. Nat. Commun. 5:3457 doi: 10.1038/ncomms4457 (2014).